Bis-silylation of internal alkynes enabled by Ni(0) catalysis 1,2-Bis-silyl alkenes have exciting synthetic potential for programmable sequential synthesis via manipulation of the two vicinal silyl groups. Transition metal-catalyzed bis-silylation of alkynes with disilanes is the most straightforward strategy to access such useful building blocks. However, this process has some limitations: (1) symmetric disilanes are frequently employed in most of the reactions to assemble two identical silyl groups, which makes chemoselective differentiation for stepwise downstream transformations difficult; (2) the main catalysts are low-valent platinum group transition metal complexes, which are expensive; and (3) internal alkynes remain challenging substrates with low inherent reactivity. Thus, the development of abundant metal-catalyzed bis-silylation of internal alkynes with unsymmetrical disilanes is of significance. Herein, we solve most of the aforementioned limitations in bis-silylation of unsaturated bonds by developing a strongly coordinating disilane reagent and a Ni(0) catalytic system. Importantly, we sufficiently realize the stepwise recognition of the two silyl groups, making this synthetic protocol of wide potential utility. The numerous applications of organosilicon compounds, ranging from organic synthetic chemistry and materials science to medicinal chemistry, indicate that the development of reliable and inexpensive methods for rapid preparation of silylated synthons is of great demand [1] , [2] , [3] , [4] , [5] . Within this context, transition metal-catalyzed bis-silylation of alkynes with disilanes, especially acyclic disilanes, has attracted substantial interest, as reflected by the ample body of literature [6] , [7] , [8] , [9] , [10] , [11] , [12] . The olefinic products juxtaposing two vicinal silicon atoms have been recognized as versatile building blocks leading to high-value scaffolds, such as densely substituted alkenes (Fig. 1a ) [13] , [14] , [15] , [16] , [17] . Despite significant advances in this reaction, there are still some limitations: (1) symmetric disilanes are frequently employed in most reactions to assemble two identical silyl groups on olefinic products, but are difficult to differentiate chemoselectively for stepwise downstream transformations [18] , [19] , [20] , [21] , [22] , [23] , [24] , [25] ; (2) the main catalysts are low-valent platinum group transition metal complexes, which are expensive; and (3) internal alkynes remain challenging substrates with low inherent reactivity in most catalytic systems. Fig. 1: Research background and our study on Ni(0)-catalyzed bis-silylation of internal alkynes with unsymmetric disilanes. a Some multi-substituted alkenes as drugs and luminogens. b The seminal report on bis-silylation of internal alkynes with acyclic disilanes (Ozawa’s work). c The breakthrough on bis-silylation of internal alkynes with stable disilanes (Spencer’s work). d Development of directing group-activated air-stable disilane for bis-silylation. e Bis-silylation of internal alkynes with air-stable disilane enabled by Ni(0) catalysis (this work). Full size image To date, only two examples of cis -bis-silylation of internal alkynes with acyclic disilanes have been reported. Ozawa and coworkers reported seminal work on the bis-silylation of internal alkynes by employing Me 3 SiSiF 2 Ph as the disilane reagent with a Pd catalyst (Fig. 1b ) [26] . However, the high toxicity, moisture sensitivity, and intolerance to various Lewis bases of Me 3 SiSiF 2 Ph, as well as the instability of the bis-silylated products (unstable on silica) severely limit the practicality of this method. In 2015, Spencer and coworkers made an important breakthrough in the intermolecular bis-silylation of internal alkynes with air-stable hexamethyldisilane by using the [(NHC) 2 Pd(SiMe 3 ) 2 ] (NHC = N-heterocyclic carbene) complex as the precatalyst (Fig. 1c ) [27] ; however, their system has two drawbacks: (1) such a bis(silyl)Pd precatalyst is relatively difficult to access and must be handled in an ampoule due to its extreme instability; (2) the two identical TMS groups on the product are inert and indistinguishable for downstream transformations. Clearly, the development of abundant metal-catalyzed bis-silylation reactions of internal alkynes with unsymmetrical disilanes is of significance and would increase the utility of this process. Recently, Song and coworkers developed an air-stable unsymmetrical disilane by attaching a coordinating group to one of the two silicon atoms, which was successfully applied to the Pd-catalyzed bis-silylation of terminal alkynes [28] . Such an unsymmetrical disilane is air-stable and offers exciting possibilities to differentiate the reactivities of the two silyl groups introduced. However, the weak coordinating ability and the intrinsic reactivity of the amide group on Song’s reagent have decreased their application scope. We envisioned that practical bis-silylation of internal alkynes with air-stable unsymmetrical disilane could be achieved by tuning the variety of directing groups on the silicon atoms and choosing appropriate transition metal catalytic systems, yielding tetrasubstituted vinylsilanes. In fact, despite the existence of numerous methods to produce vinylsilanes [29] , [30] , [31] , the synthesis of tetrasubstituted vinylsilanes remains challenging [32] , [33] , [34] , [35] . Inspired by the strong coordination ability of N-heterocycles that enables the formation of thermodynamically stable metallacycles [36] , we wondered whether the introduction of a quinolyl group on a disilane would change the coordinating ability of the metal center and result in higher reactivity. Herein, we achieve the bis-silylation of internal alkynes with an air-stable unsymmetrical disilane by developing a strongly coordinating disilane reagent 8-(2-substituted-1,1,2,2-tetramethyldisilanyl)quinoline (TMDQ) and a Ni(0)-catalytic system (Fig. 1c ). Notably, Ni(0) catalysis has never been utilized in the bis-silylation of π-bonds with acyclic disilanes before [37] , [38] . Moreover, both the disilane reagent and the products in our study are stable on silica, and the reactivities of the two nonequivalent silyl groups on the olefinic products can be distinguished sufficiently, making this synthetic protocol of great potential utility. Preparation of strongly coordinating disilane TMDQ reagents TMDQ reagents were easily synthesized in one step, as shown in Fig. 2 . With commercially available, inexpensive 8-bromoquinoline as the starting material, the lithium halogen exchange reaction with sec -butyllithium followed by the treatment with Me 2 RSiSiMe 2 Cl yielded the strongly coordinating disilane TMDQ reagents 1a–d . Notably, our TMDQ reagents are air-stable, colorless liquids that can be synthesized practically on the gram scale and can be easily purified by column chromatography. Fig. 2: The synthetic route for producing the strongly coordinating disilane TMDQ reagent. The detailed procedures for preparation of these disilane TMDQ reagents have been presented in Supplementary Information (SI). 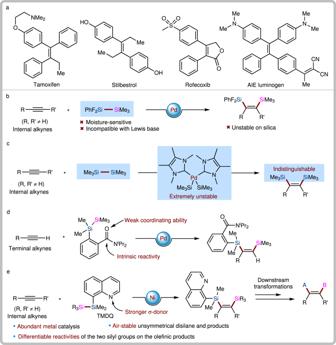Fig. 1: Research background and our study on Ni(0)-catalyzed bis-silylation of internal alkynes with unsymmetric disilanes. aSome multi-substituted alkenes as drugs and luminogens.bThe seminal report on bis-silylation of internal alkynes with acyclic disilanes (Ozawa’s work).cThe breakthrough on bis-silylation of internal alkynes with stable disilanes (Spencer’s work).dDevelopment of directing group-activated air-stable disilane for bis-silylation.eBis-silylation of internal alkynes with air-stable disilane enabled by Ni(0) catalysis (this work). Full size image Condition screening With the unsymmetrical disilane TMDQ reagent in hand, we conducted the reaction of disilane 1a and diphenyl acetylene 2a under the Pd-catalyzed conditions reported by Song and coworkers for the bis-silylation of terminal alkynes [28] , but these reagents were found to be completely unreactive under these conditions (Table 1 , entry 1). After numerous attempts to optimize the reaction conditions (for more details, see Supplementary Table 1 in Supplementary Information), we found that the bis-silylation of unsymmetrical disilane 1a and diphenyl acetylene 2a occurred smoothly under Ni(0)-catalytic conditions, and the optimized conditions were 10 mol % Ni(COD) 2 , SIPr (12 mol%), and toluene as the solvent to produce cis -bis-silylated olefinic product 3aa in 98% yield at 100 °C for 24 h (Table 1 , entry 2). To confirm the structure of 3aa , structural analysis of a single crystal was carried out by X-ray diffraction. Control experiments were subsequently carried out to investigate the effect of each component. The use of SIPr generated in situ from SIPr·HCl incorporation of t- BuOK led to inferior yield (entry 3). Switching the SIPr·HCl to ICy·HBF 4 dramatically decreased the yield of this reaction (entry 4). Reducing the amount of the Ni catalyst to 5 mol% resulted in a slightly decreased yield (entry 5). Interestingly, the bis-silylation reaction also proceeded smoothly, with 92% yield, when Ni(COD) 2 /PPh 3 was used as the catalytic system (entry 6). We also investigated the effects of disilane reagents on this bis-silylation reaction under the optimized conditions. We found that no reaction occurred if unsymmetric disilane 1a was replaced with Me 3 SiSiMe 3 ( 1e ) under the optimized conditions (entry 7). No desired bis-silylated product was detected if the 8-quinolinyl group was replaced with a 1-naphthalenyl group in unsymmetric disilane 1a (entry 8). Notably, the reaction occurred, albeit at a low yield, when Song’s disilane reagent 1g was used during the reaction (entry 9). These results indicate that the introduction of the directing group on the unsymmetric disilane was vital for ensuring this bis-silylation reaction. Table 1 Control experiments for the screening of reaction condition. 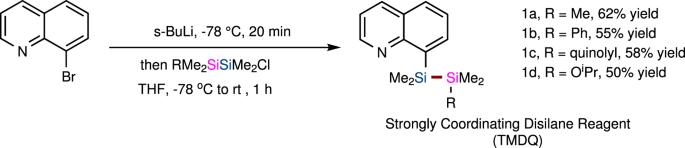Fig. 2: The synthetic route for producing the strongly coordinating disilane TMDQ reagent. The detailed procedures for preparation of these disilane TMDQ reagents have been presented inSupplementary Information(SI). Full size table Substrate scope We next investigated the scope of unsaturated substrates and TMDQ reagents for this bis-silylation (Table 2 ). We found that PPh 3 as the ligand in the model reaction resulted in good yield, and the other internal alkynes generally gave the bis-silylated products in low to moderate yields. To our delight, the reaction of TMDQ reagent 1a and a wide variety of symmetric para- or meta -substituted diaryl alkynes with different electronic properties afforded the desired products in good to excellent yields with exclusive cis -selectivity ( 3ab – al ) by use of SIPr as the ligand. Multi-substituted diaryl alkynes also provided the corresponding bis-silylated products in high yields ( 3am − an ). Naphthalene-substituted alkynes could also successfully react with the TMDQ reagent to deliver bis-silylated olefins ( 3ao − ap ). Importantly, this method was remarkably tolerant of various important functional groups on the phenyl ring of diaryl alkynes, such as F, CF 3 , COOEt, and OMe groups. Next, various symmetrical aliphatic alkynes were evaluated. We found that using 2-dicyclohexylphosphino-2′,6′-dimethoxybiphenyl (Sphos) as the ligand resulted in high yields with a low catalyst loading under milder reaction conditions ( 3aq – at ). Furthermore, the electron-withdrawing internal alkyne dimethyl acetylenedicarboxylate as the substrate was also subjected to Ni-catalytic conditions. Unfortunately, it proved unreactive. In addition, the other TMDQ reagents produced from 8-bromoquinoline were also competent coupling partners, enabling access to the corresponding bis-silylated olefinic products ( 3ba − da ). In addition to symmetrical alkynes, unsymmetrical internal alkynes were also investigated. Unfortunately, 1-phenylpropyne was inert under Ni-catalyzed standard conditions. To ensure reactivity and the regioisomeric ratio, we further screened a large set of reaction parameters, such as ligands, solvents, and disilane reagents, as shown in Supplementary Tables 2 and 3 in the Supplementary Information. Finally, disilylated product 3au was obtained in 82% yield at 83:17 r.r., when BrettPhos was used as the ligand and DMF was used as the solvent. Moreover, we found that employment of TMDQ 1d as the disilane reagent during the reaction further increased the regioisomeric ratio to 86:14 ( 3du in Table 2 ). Then, diverse aryl methyl acetylenes were evaluated under the modified conditions. In general, the aryl substituent with different electronic properties did not influence the yield or the regioisomeric ratio, generally giving the corresponding products ( 3du – dz ) in good yields with good regioselectivities (up to 9:1). 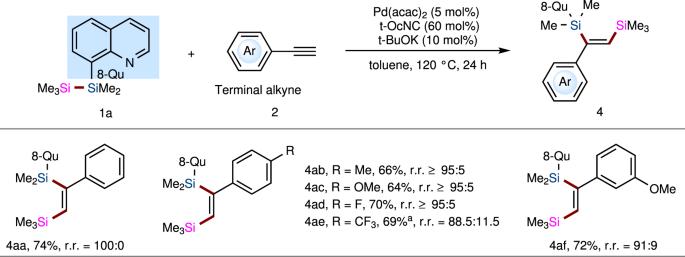Fig. 3: The bis-silylation reaction of TMDQ reagent 1 with terminal alkyne 2. Standard reaction conditions: disilane1a(52 mg, 0.2 mmol), terminal alkyne2(41 mg, 44 μL, 0.4 mmol), Pd(acac)2(3 mg, 0.01 mmol),t-OcNC (17 mg, 0.12 mmol), andt-BuOK (2.3 mg, 0.02 mmol) in toluene (2 mL) at 120 °C under N2atmosphere for 24 h. SeeSupplementary Information(SI) for details. Phenyl propyl acetylene was also a suitable substrate, affording 3dä in 65% yield with 73% regioselectivity. Notably, these two regioisomers were separable by column chromatography, which increases the practicality of this method. The structure of the major isomer was confirmed by X-ray crystal diffraction analysis of compound 3dz . Table 2 Substrate scope. Full size table Following the success of Ni-catalyzed bis-silylation of internal alkynes with diverse TMDQ reagents, we proceeded to examine the terminal alkyne as the coupling partner. Unfortunately, in the optimized Ni-catalytic system, the reaction of TMDQ reagent 1a and phenylacetylene did not proceed. Presumably, it might be because terminal alkynes are generally more active than internal alkynes and feasible to coordinate with the metal center more tightly by forming the Ni/alkyne (1:2) complex, leading to catalyst deactivation. Inspired by the Pd-catalytic system developed by Song, we replaced the Ni catalyst with a Pd-catalytic system for this reaction. After extensive screening, we found that the reaction of unsymmetric disilane 1a with terminal phenylacetylene proceeded smoothly with Pd(acac) 2 (5 mol%), tert -octylisocyanide ( t -OcNC, 6 mol%), and t- BuOK (10 mol%) in toluene for 24 h at 120 °C, affording desired bis-silylated product 4aa in 74% yield with complete regioselectivity (100:0 r.r.). Then, several aryl acetylenes were further tested for the bis-silylation reaction with TMDQ reagent 1a , affording the corresponding products 4ab – af (Fig. 3 ). Alkyl acetylene was unreactive. 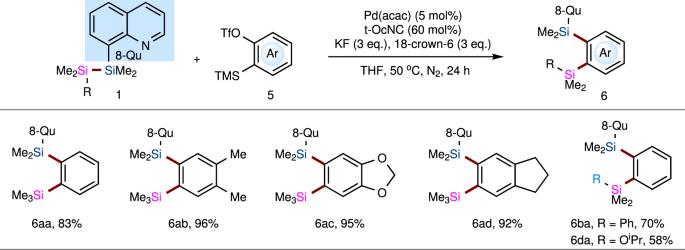Fig. 4: The bis-silylation reaction of TMDQ reagent 1 with aryne 5. Standard reaction conditions: TMDQ reagent1(0.2 mmol), aryne precursor5(0.4 mmol), Pd(acac)2(3 mg, 0.01 mmol),t-OcNC (17 mg, 0.12 mmol), KF (35 mg, 0.6 mmol), and 18-crown-6 (159 mg, 0.6 mmol) in THF (2 mL) at 50 °C under N2atmosphere for 24 h. See Supplementary Information (SI) for details. In general, our TMDQ reagent led to low yields and comparable regioselectivity relative to Song’s system for the bis-silylation reaction of terminal alkynes. Fig. 3: The bis-silylation reaction of TMDQ reagent 1 with terminal alkyne 2. Standard reaction conditions: disilane 1a (52 mg, 0.2 mmol), terminal alkyne 2 (41 mg, 44 μL, 0.4 mmol), Pd(acac) 2 (3 mg, 0.01 mmol), t -OcNC (17 mg, 0.12 mmol), and t -BuOK (2.3 mg, 0.02 mmol) in toluene (2 mL) at 120 °C under N 2 atmosphere for 24 h. See Supplementary Information (SI) for details. Full size image The importance of arynes as useful reactive intermediates undergoing a wide variety of reactions has been well illustrated [39] , [40] , [41] . For example, in 2003, Yoshida and Kunai disclosed the palladium-catalyzed bis-silylation of arynes with strained cyclic disilanes [42] , which afforded diverse benzoannulated disilacarbocycles. However, until now, no report has been published on the addition of an acyclic disilane to arynes, which is an excellent and straightforward way to synthesize 1,2-disilyl-substituted benzenes that have been widely employed as starting materials for preparing diverse reagents and π-building blocks [43] , [44] , [45] , [46] . Following the success of the bis-silylation of internal and terminal alkynes with the TMDQ reagent, we set out to explore the application of this reagent in the bis-silylation of arynes to access 1,2-disilylbenzene derivatives that are usually obtained via the reaction of 1,2-dichlorobenzenes or 1,2-dibromobenzenes with chlorosilanes [47] , [48] , [49] . We investigated the reaction of TMDQ 1a and an aryne generated in situ from 2-(trimethylsilyl)aryl triflate ( 5a ) and a fluoride ion (KF/18-crown-6). However, no desired product was detected under the Ni-catalytic system. 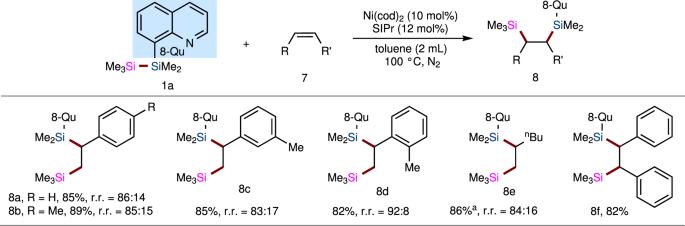Fig. 5: The bis-silylation reaction of TMDQ reagent 1a with alkenes 7. Standard reaction conditions: the mixture of Ni(COD)2(5.6 mg, 0.02 mmol) and SIPr (9.5 mg, 0.024 mmol) in toluene (2 mL) was stirred for 30 min, then disilane reagent1(0.2 mmol) and specific alkene7(0.4–2 mmol) were added. The reaction was heated to 100 °C with vigorous stirring for 48 h under N2atmosphere. See Supplementary Information (SI) for details.a10.0 equiv alkene was used. To our delight, the screening results showed that desired product 6aa was obtained in 83% yield when the Pd-catalytic system was used (Supplementary Table 5 in Supplementary Information). We continued our studies by investigating the scope with respect to the aryne components (Fig. 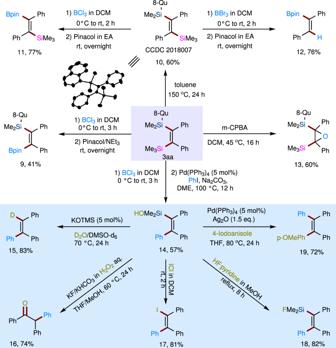Fig. 6: Synthetic utilities of product 3aa. The product3aaresulting from bis-silylation can be conveniently transformed to a variety of skeletons by programmable sequential synthesis. Yields are for isolated and purified products. The detailed procedures for these downstream transformations have been presented in Supplementary Information (SI). 4 ). The reaction of symmetric arynes with TMDQ reagent 1a provided desired products 6aa – ad in excellent yields. Moreover, TMDQ reagent 1d also reacted smoothly with benzyne to produce 1,2-disilyl-substituted benzene 6da in 58% yield. Fig. 4: The bis-silylation reaction of TMDQ reagent 1 with aryne 5. Standard reaction conditions: TMDQ reagent 1 (0.2 mmol), aryne precursor 5 (0.4 mmol), Pd(acac) 2 (3 mg, 0.01 mmol), t -OcNC (17 mg, 0.12 mmol), KF (35 mg, 0.6 mmol), and 18-crown-6 (159 mg, 0.6 mmol) in THF (2 mL) at 50 °C under N 2 atmosphere for 24 h. See Supplementary Information (SI) for details. Full size image In addition to diverse alkynes, alkenes as substrates for bis-silylation with our disilane reagent 1a have also been tested under Ni-catalyzed and Pd-catalyzed conditions. In fact, transition metal-catalyzed intermolecular bis-silylation is still a challenge. Generally, conjugated or strained double bonds are needed to ensure reactivity. After a few attempts at the reaction of 1a with styrene 7a , we found that the Pd catalyst was unreactive. In contrast, styrene 7a successfully reacted with disilane 1a in the Ni 0 -catalyzed reaction to afford the corresponding bis-silylated product 8a in 85% yield and with a 86:14 regioisomeric ratio (Fig. 5 ). Next, we carried out the nickel-catalyzed bis-silylation of diverse alkenes with 1a . First, all of the reactions with substrates bearing a substituent in the para -, meta -, or ortho -position proceeded well with good yields and regioselectivities ( 8b–d ). Likewise, the reaction also proceeded well with 1-hexene, affording bis-silylated product 8e in 86% yield and with 84:16 regioselectivity. Moreover, the scope of the reaction could be further extended to cis -bisaryl alkene ( 8f ). However, cis -bisalkyl alkenes and trans -alkenes are currently not suitable under the optimized conditions. Fig. 5: The bis-silylation reaction of TMDQ reagent 1a with alkenes 7. Standard reaction conditions: the mixture of Ni(COD) 2 (5.6 mg, 0.02 mmol) and SIPr (9.5 mg, 0.024 mmol) in toluene (2 mL) was stirred for 30 min, then disilane reagent 1 (0.2 mmol) and specific alkene 7 (0.4–2 mmol) were added. The reaction was heated to 100 °C with vigorous stirring for 48 h under N 2 atmosphere. See Supplementary Information (SI) for details. a 10.0 equiv alkene was used. Full size image Synthetic utility Notably, all of these bis-silylated products are air-stable, can react on a gram scale and are easily purified on a silica column (1.18 g of 3aa , 90%). To investigate the synthetic utility of the olefinic products obtained by our method, we took 3aa as an example to prove that the two vicinal silyl substituents could be sufficiently differentiated in downstream transformations to achieve structurally diverse skeletons (Fig. 6 ). The TMS group on product 3aa could be chemoselectively transformed to a Bpin group by treatment with BCl 3 in DCM, followed by quenching with Pinacol at room temperature, yielding compound 9 . Treatment of 3aa in toluene at 150 °C for 24 h led to cis -to- trans isomerization of the two vicinal silyl groups to yield product 10 in 60% yield, which was confirmed by X-ray crystal analysis. In contrast, the 8-QuMe 2 Si moiety on trans -product 10 preferentially reacted with BCl 3 in DCM to yield compound 11 , in which the TMS group remained intact. Interestingly, by employing BBr 3 in DCM, both desilylation and borylation of product 10 took place to afford tri-substituted alkenylborate 12 in 76% yield. In addition, cis -epoxidation of the C=C bond of 3aa afforded product 13 in 60% yield by treatment with m -CPBA in DCM. Of note, because of the distinguishable reactivities of the two nonequivalent silyl groups on 3aa , this compound could be utilized as a platform to regio- and stereoselectively transform into diverse tetrasubstituted olefins in a stepwise manner by a sequential assembly strategy. Triaryl-substituted alkenylsilanol 14 was first synthesized from 3aa by sequential borodesilylation and Suzuki coupling. Then, the remaining Me 2 SiOH group on 14 originating from hydrolysis of the 8-Qu group during Suzuki coupling could further undergo diverse transformations, such as deuteration, Tamao’s oxidation, iodination, and fluorination, to achieve structurally diverse synthetic building blocks 15 , 16 , 17 , and 18 , respectively. Furthermore, the Hiyama−Denmark cross-coupling of 14 and 4-iodoanisole proceeded smoothly to give tetraaryl-substituted olefin 19 in 72% yield, which has been widely used as an AIE luminogen. Fig. 6: Synthetic utilities of product 3aa. The product 3aa resulting from bis-silylation can be conveniently transformed to a variety of skeletons by programmable sequential synthesis. Yields are for isolated and purified products. The detailed procedures for these downstream transformations have been presented in Supplementary Information (SI). Full size image The introduction of an alkoxy group attached to silicon generally modifies the reactivity of the corresponding silyl group. Thus, we wondered whether our product 3da bearing an isopropoxy group on the silicon atom possesses richer and more colorful reactivities than compound 3aa (Fig. 7 ). Indeed, there is no need for preborodesilylation for the cross-coupling of 3da with aryl electrophiles. We show the cross-coupling of 3da with benzoic anhydride to afford compound 20 under Rh I -catalytic conditions. The Si–O bond of product 3da can be reduced by LiAlH 4 to give the corresponding hydrosilane 21 (70% yield), which can further serve as an indispensable reagent in hydrosilylation. In addition, 3da can also be easily hydrolyzed to yield the corresponding silanol 22 in 71% yield, which is also capable of cross-coupling with iodobenzene to produce compound 23 and cyclization to obtain compound 24 in 97% yield, which was synthesized by Au-catalyzed dehydrogenative cycloaddition of specific dihydrodisilanes to alkynes. Fig. 7: Synthetic utility of product 3da. These results indicate that the two vicinal silyl substituents on product 3da can be sufficiently differentiated in downstream transformations to achieve structurally diverse skeletons. Yields are for isolated and purified products. The detailed procedures for these downstream transformations have been presented in Supplementary Information (SI). Full size image Proposed mechanism Following the literature, we proposed a catalytic cycle for our study that begins with coordination of Ni 0 to the nitrogen atom of disilane reagent 1a to form intermediate A , which is followed by coordination-assisted oxidative addition of Si−Si bonds [50] , [51] , [52] , thus producing metallacycle B (Fig. 8 , path A). Complex B further undergoes an intermolecular silylmetalation of an internal alkyne to deliver intermediate C , followed by reductive elimination to afford bis-silylated product 3 and regenerate the Ni 0 catalyst. 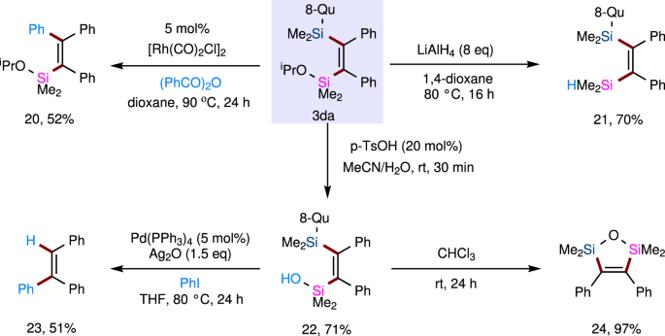Fig. 7: Synthetic utility of product 3da. These results indicate that the two vicinal silyl substituents on product3dacan be sufficiently differentiated in downstream transformations to achieve structurally diverse skeletons. Yields are for isolated and purified products. The detailed procedures for these downstream transformations have been presented in Supplementary Information (SI). 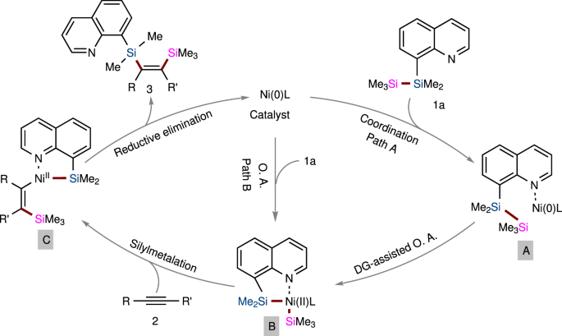Fig. 8: Proposed catalytic cycle. Specifically,A: transition state by coordination of Ni0to the nitrogen atom of disilane TMDQ reagent;B: transition state after oxidative addition of Si−Si bond;C: transition state for silylmetalation of an internal alkyne. However, other proposals, such as Si−Si oxidative addition of the Ni(0) catalyst directly, followed by coordination of the N atom on the 8-Qu group to form intermediate B (Fig. 8 , path B), cannot be ruled out at this stage. Fig. 8: Proposed catalytic cycle. Specifically, A : transition state by coordination of Ni 0 to the nitrogen atom of disilane TMDQ reagent; B : transition state after oxidative addition of Si−Si bond; C : transition state for silylmetalation of an internal alkyne. Full size image In summary, we have developed an air-stable, strongly coordinating unsymmetrical disilane reagent, TMDQ, which is capable of bis-silylation of internal alkynes in a Ni 0 -catalytic system, leading to the synthesis of bis-silylated olefinic products, in which the two nonequivalent silyl groups can be sufficiently differentiated and transformed in a stepwise manner for further downstream transformations, making this synthetic protocol of great potential utility. The introduction of the 8-Qu group on the silicon atom at the unsymmetrical disilane and employment of a Ni(0)-catalytic system are crucial for adjusting the coordinating ability of the metal center and achieving higher reactivity. General procedure for Ni-catalyzed bis-silylation of internal alkynes with TMDQ reagent In the nitrogen-filled glovebox, to an oven-dried 8-mL sealed tube equipped with a Teflon-coated magnetic stir bar were added Ni(COD) 2 (5–10.0 mol%), ligand (10–12.0 mol%), toluene (2 mL), and the reaction mixture was stirred for 30 min, then TMDQ reagent 1 (0.2 mmol, 1.0 equiv. ), internal alkynes 2 (0.4–2 mmol, 2.0–10 equiv.) were added. The vial was sealed with a screw-top septum cap, removed from the glovebox and placed in a heating block that was preheated to 100 °C with vigorous stirring for 36–48 h under N 2 atmosphere. After been cooled to room temperature, the reaction mixture was filtered through a pad of celite and concentrated in vacuo. The resulting residue was purified by silica gel flash chromatography to give the desired product 3 .